Electrochemical tunnelling sensors and their potential applications Electrochemical sensors based on measuring the tunnelling current across nanoscale electrode junctions in solution are emerging as a new class of single-molecule sensors. They combine extremely high spatial resolution with sensitivity to the electronic structure of the analyte. This opens up perspectives towards the label-free detection of small molecules, the characterization of catalytic or enzymatic processes at the single-molecule level as well as the analysis of biopolymers with sub-molecular resolution, Fig. 1 . To this end, label-free, fast and inexpensive RNA and DNA sequencing may be in reach, potentially revolutionizing the way we perform gene sequencing today. 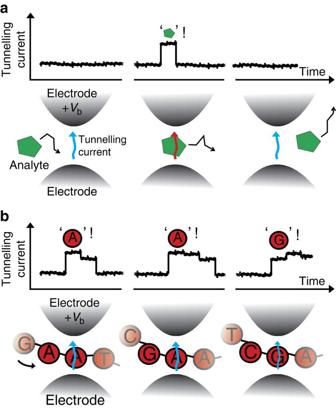Figure 1: Probing dynamic processes at the solid/liquid interface by tunnelling. (a) Sensing of a freely diffusing analyte that first diffuses into the tunnelling junction, then bridges the gap and finally detaches and diffuses out of the junction. (b) Tunnelling readout of DNA base composition. In this scenario, the DNA strand moves along the tunnelling junction in a controlled conformation and at well-defined speed. Each base interacts with the tunnelling junction and is identified by a characteristic tunnelling conductance.Vbis the bias voltage applied to the two tunnelling electrodes. Figure 1: Probing dynamic processes at the solid/liquid interface by tunnelling. ( a ) Sensing of a freely diffusing analyte that first diffuses into the tunnelling junction, then bridges the gap and finally detaches and diffuses out of the junction. ( b ) Tunnelling readout of DNA base composition. In this scenario, the DNA strand moves along the tunnelling junction in a controlled conformation and at well-defined speed. Each base interacts with the tunnelling junction and is identified by a characteristic tunnelling conductance. V b is the bias voltage applied to the two tunnelling electrodes. Full size image Charge transfer by quantum-mechanical tunnelling is one of the most ubiquitous elementary processes in nature and features in areas as diverse as electron or hydrogen transfer in enzymatic reactions, interfacial charge transfer at metal electrodes in solution, thin-layer devices in electronics, charge transfer between crystal defects and radioactive α-decay [1] . Important applications exploiting tunnelling transport include the Esaki tunnelling diode and the scanning tunnelling microscope (STM)—both recognized with the Nobel Prize in Physics for their inventors, namely Esaki in 1973 (jointly with Josephson), and Binnig and Rohrer in 1986, respectively. 'Tunnelling' refers to the transport of electrons (or other light charge carriers) across a nanometre-sized gap, a molecule or even an insulating layer between two electrodes. Upon application of a bias voltage V bias between the two electrodes, negatively charged electrons are more likely to be transported towards the positively biased electrode and a so-called 'tunnelling current' I t is detected. The latter depends exponentially on gap size, which is the reason for the high spatial resolution of STM, the applied voltage V b and the electronic structure of the medium in the gap. To this end, the electrode junction may be represented by a transmission function that characterizes the probability of electrons moving from one electrode across the gap into the second electrode, summarized over all energy levels. Hence, the more accessible the energy levels in the junction, and the better their electronic coupling to the electrodes, the higher current across the junction. This also implies that the tunnelling current is sensitive to the immediate molecular environment of the bridge as well as any dynamic effects (molecular reorganization and chemical modification). Box 1 gives a brief introduction and also includes a short tutorial on how to calculate the transmission function using Green's functional theory. The interested reader is referred to specialist reviews and textbooks for further details [2] , [3] , [4] , [5] . The focus of this review is on how tunnelling detection could be used as a new and unique sensor concept. Tunnelling charge transport in liquid environments is discussed, highlighting a number of distinctive features, for example the effect of environmental dynamics and of small-molecule binding to the tunnelling junction. This leads to the notion of catalytically modulated tunnelling as a new way of studying enzyme kinetics at the single-molecule level. Electrochemical tunnelling sensors are considered as a tool for label-free structural analysis of large biopolymers with sub-molecular resolution, for example for DNA sequence analysis or the detection of epigenetic markers. Box 1: Some theoretical aspects of charge transport in molecular junctions. Charge transport across an electrode/molecule/electrode junction is illustrated in the adjacent figure: The two electrodes 1 and 2 have Fermi levels μ 1,2 , which differ by − eV b . The molecular energy level is coupled to the electrode leads by h 0 and broadened in energy by an amount γ . The corresponding Fermi functions and their difference, according to equation (2), are shown on the right-hand side. In the coherent limit of charge transport, there is no energy exchange between the tunnelling electrons and their surroundings in the junction—the phase is preserved. This is usually the case if the junction is short and well coupled to the electrode leads. γ is large and the electronic states strongly delocalized. According to the uncertainty principle, γ ·τ ≥ ħ, the lifetime τ of the electronic state is small, because an electron can more easily 'escape' into the leads. If tunnelling electrons do exchange energy during the process, for example, by exciting molecular vibrations or phonons on the bridge, incoherent tunnelling occurs; the phase is then not preserved. Ultimately, in the case of strong coupling to the nuclear environment on the bridge, which is typical of solution environments, tunnelling electrons may be trapped on particular sites in the junction. The transport process is then composed of a sequence of individual, thermally activated charge transfer steps (hopping), each with a characteristic rate constant. Charge hopping is usually dominant for long, weakly coupled molecular junctions, because the distance dependence is weaker than in coherent tunnelling ( d −1 versus e −d ). In general, however, it is not a priori clear, which mechanism is at hand in a given situation. The transition from to one to the other may be dependent on subtle structural details of the junction, for example the binding to electrode surface or the molecular conformation (which is time dependent). The interested reader is referred to specialist textbooks and reviews on the subject for further details [3] , [5] . Returning to the coherent limit as the arguably simplest charge transport mechanism, the observed net current I t is the difference between electron flow from electrode 1 to electrode 2 and vice versa [5] . The flux depends on the Fermi distribution of each 'source' of electrons, f 1 ( E ) and f 2 ( E ), respectively, and a transmission function T ( E ) characterizing the junction itself. As all energy levels contribute to some degree, the total current is obtained by integrating over all energies: Equation (2) establishes a direct relation between the current, and ultimately the conductance, and the transmission function; a concept first derived by Landauer using scattering theory. Note that μ 2 = μ 1 + qV b ( q : charge), and f 2 ( E )=[1+exp( E −( μ 1 + q · V b )/( k B · T )] −1 ; I t is non-zero when V ≠0. f 1 ( E )− f 2 ( E ) is largest for E ≈ μ 1,2 . This means that energy levels close to the Fermi energies μ 1,2 are most efficient in transporting charge. Formally, the transmission function T ( E ) maybe calculated using the Green's functional formalism, where 'tr' is the trace of the subsequent matrix and A 1,2 the spectral functions, that is, the matrix version of the density-of-state curve for a single level multiplied by 2π. Γ 1,2 is the broadening matrix of the electrodes 1 and 2 (the multi-level equivalent of γ for each electrode). It is defined in terms of the self energies Σ 1,2 , which characterize the effect of the reservoirs on the channel: Γ 1,2 =i( Σ 1,2 − Σ 1,2 + ). The superscript '+' refers to the conjugate transpose; G and G + are the retarded and the advanced Green's function of the junction. I is the identity matrix, 0 + a small energy term related to the energy broadening of each state and H the Hamiltonian of the bridge. G thus contains the 'molecular' information. Taking a single channel of length d coupled to two electrodes 1 and 2 with an energy h 0 as a simple model system (see chapter 9 of ref. 5 ), all matrices H , Σ and so on, are reduced to scalars: E c is the energy of the conduction band edge, U 0 / d is an additional potential acting on the channel, and k is the wave vector of the electron. The energy E is related to k via the dispersion relation Note that the velocity v of the electron as a function of k is given by The broadening 'matrices' are then given by Γ 1,2 = h̄ħv / L , equations (6) and (8). The retarded and advanced Green's functions are obtained by combining equations (5), (6), (7) in equation (4) ( i 0+→0), yielding respectively. As G , G + and Γ 1,2 are scalar values, the trace in equation (3) reduces to a simple product. The transmission function is calculated to give: For large U 0 , T ( E ) becomes very small and the current mediated by the molecular level is zero. If U 0 =0 (perfect alignment of the levels), then T ( E )≈1. The Fermi functions may be replaced by step functions, if thermal broadening is small enough, implying that f 1 − f 2 =1 between μ 1 and μ 2 (and zero elsewhere). Taking into account that each level may carry two electrons of opposite spin, the conductance quantum is given by Note that there may still be tunnelling barriers, for example at the contacts. However, under resonant conditions, their exact nature does not affect the channel conductance. Tunnelling is not restricted to any particular state-of-matter and occurs through thin insulating (solid) films, vacuum, air and even solution environments. In fact, it was already in 1931 that Gurney [6] recognized the significance of quantum mechanical tunnelling for electrochemical reactions at metal electrodes. The STM is now routinely used in solution, including aqueous electrolytes, organic solvents and ionic liquids (ILs) [7] , [8] . Exactly how electrons tunnel through liquid-filled electrode junctions is not a trivial matter and only carefully conducted experiments in combination with theory and simulations has finally led to a better understanding of the processes involved. One would expect the molecular structure of the bridge to change with time, and that potentially more than one bonding pattern bridges the electrode gap at any given moment. It is therefore convenient to represent the tunnelling medium by an effective tunnelling barrier Φ B , which combines all these more subtle effects and is easily determined experimentally from tunnelling current-distance spectroscopy in STM. Compared with vacuum, the experimentally measured tunnelling barriers in water-filled junctions are significantly reduced. While tunnelling barriers in vacuum are usually in the 4–5-eV range, depending on the work function of the electrode material used, the corresponding values in aqueous solution drop to about 1–2 eV (refs 9 , 10 , 11 , 12 , 13 ). This is at least in part due to image charge effects, the local ion distribution and solvent polarization, and results in an increase of the effective tunnelling distance by roughly a factor of two for the barrier values given above [14] , [15] . In line with this more complex picture, Nitzan et al . suggested that trap states associated with cavities in the water structure may provide transient, very short-lived resonances ( ∼ 10 fs) lowering the apparent barrier height [16] . Moreover, based on molecular dynamics/NEGF calculations, Negre et al . [17] found that particular water configurations can mediate charge transport via hydrogen-bonding networks; a finding that echoes Beratan's [18] suggestion about hydrogen-bond-mediated electron transfer in proteins. The tunnelling current displays a non-exponential dependence on gap size, depending on the ion distribution at the solid/liquid interface [11] , [13] , [19] , [20] . Hugelmann and Schindler found an oscillatory substructure in the tunnelling barrier that most likely reflects the ion distribution at the solid/liquid interface; a view that was later confirmed by Jacob and Kolb using STM studies combined with DFT calculations. [10] , [21] It is instructive to consider the different time scales of the processes involved. The characteristic time associated with the tunnelling process is on the order of 10 fs (ref. 22 ), which is similar to the lifetime of the proposed resonant cavity structures mentioned above [16] . Transient formation of hydrogen bond networks, acting as an intermittent molecular bridge, and dynamic effects in covalently attached molecular 'wires' occur in the picosecond to nanosecond range [17] , [18] , [23] , [24] ; this is still too fast to be resolved directly in a low-current measurement. On the other hand, other dynamic effects leading to tunnelling current modulation occur on a much slower timescale and include intermittent 'electron trapping' in polar solution environments, giving rise to characteristic noise features [25] and molecular binding events in the electrode junction. The latter could be exploited for studying interfacial catalytic or enzymatic processes on the single-molecule level [26] , [27] , [28] , catalytic activity mapping on the surface or for stochastic sensing of analyte molecules in solution, vide infra . Faradaic processes on the electrode surface, such as oxidation or reduction of molecules in solution, can result in currents much larger than the tunnelling current and thus dominate the detected signal. Such electrochemical reactions have, however, little 'diagnostic' value in the present context and need to be minimized, for example by reducing the surface reactivity or the electrochemically active surface area. 'Redox cycling' is a process where a molecule is first oxidized on one electrode, then diffuses or migrates to the second electrode in close proximity, where it is then reduced. The cycle is completed by renewed oxidation on the first electrode and so forth. This is well known in SECM (scanning electrochemical microscopy) and used as a mechanism to control the distance between SECM probe and substrate surface [29] . At very small electrode distances, this can result in measurable steady-state currents, involving a few or even a single molecule(s) [30] , [31] . Such redox cycling may easily be mistaken for (redox-mediated) hopping transport and one expects that for sufficiently small electrode distances, the two scenarios in fact converge, namely when the mass transport resistance becomes negligible compared with the charge transfer resistances at the respective electrode interface. Given the sensitivity of the tunnelling current to local electrostatic and bonding interactions, it is clear that solution environments offer a range of opportunities towards tunnelling-based analysis of interfacial processes. From an application point of view, there are other features: Liquid environments offer increased flexibility with regards to sample handling and preparation, particularly for large biomolecules such as proteins and DNA. This may include lab-on-a-chip technologies, but also manipulating their three-dimensional structure, for example by chemically induced unfolding. Detection of switching events by tunnelling current modulation may be easier than measuring the corresponding Faradaic processes directly. The transient oxidation or reduction of a single redox catalyst molecule on the surface typically only involves one or two electrons. If the characteristic timescale is 1 μs, this leads to extremely small currents on the order of 100 fA, which are undetectable given the required bandwidth and potential other sources of background currents. On the other hand, the characteristic tunnelling time is much faster, say 10 fs [22] , [32] , leading to a current of 10 pA during the same time, which may be achievable using customized electronics [33] . Solution environments can enhance the stability of nanoscale electrode junctions by saturating open valences on the electrode surface, thus reducing the driving force for the electrode gap to collapse, and improve heat transfer away from the junction. The sensitivity of the tunnelling current to the electronic structure of the analyte molecule reduces or may even remove the need for additional labelling. This is required in other approaches to single-molecule sensing, such as fluorescence spectroscopy, contributing significantly to the overall operating costs. Combined with the unprecedented spatial resolution, this may provide routes towards the compositional analysis of large polymeric molecules using tunnelling currents. In fact, suggestions to use an STM for DNA sequencing were made in the 1980s and 1990s [34] , [35] , [36] , even though STM per se is a relatively slow technique and not suitable for high-throughput DNA sequencing, see below. Interfacial processes, such as surface diffusion, molecular reorientation and molecular binding events, can be detected by measuring the tunnelling current [37] , [38] , [39] , [40] , [41] . These considerations form the basis of various methods for determining the conductance of individual molecules in single-molecule electronics research [42] . The formation (or rupture) of a molecular bridge between the two electrodes is detected by an instantaneous increase (or decrease) of the tunnelling current. After recording and statistical analysis of many such events, the conductance distribution, including the mean and width, can be extracted. Interestingly in the present context, both parameters are known to depend on details of the molecule/surface bond at the atomic level and not only on the electronic properties and geometry of the bridge itself [43] , [44] . The relation between molecular binding and current modulation is, however, not always trivial. It appears that the former can cause complex current burst characteristics, which in turn contain valuable information about the molecular process itself, for example, hydrogen-bonding patterns (recognition tunnelling) [45] , [46] . Lindsay et al . distinguish between the 'tethered pair' configuration where chemical recognition occurs between surface modifiers (chemical adapters) on each electrode [47] , [48] and the 'free-analyte' configuration where a freely diffusing analyte bridge binds to each adapter at the same time, thus bridging the tunnelling gap. In both cases, recognition events result in distinct and well-defined modulation of the tunnelling current, in terms of magnitude, event frequency and other details of the tunnelling noise. Statistical analysis is then used to identify a given analyte. At present, most of this work is directed to the differentiation of DNA bases and DNA sequencing-by-tunnelling. Features of stochastic switching were also found in STM imaging and in tunnelling (distance) spectroscopy [49] , [50] : In the latter case, the STM tip is approached towards an Au-nanoparticle-modified platinum surface, immersed in an aqueous electrolyte. The tunnelling current remains low while the tip is far away from the electrode surface, then starts to oscillate between two states, which most likely correspond to the open (non-contact) and the closed (contact) states, Fig. 2 . At sufficiently small tip/surface distance, the oscillation stops and the 'closed' configuration is adopted permanently. Bistability and hysteresis in a single-molecule junction was also observed by Riel and coworkers [51] for dinitro oligophenylene–ethynylene derivatives, whereas analogues without nitro substituents did not exhibit any switching behaviour. This links the occurrence of switching events to a molecular characteristic, but again the exact nature of the 'on' state remains under debate [52] . 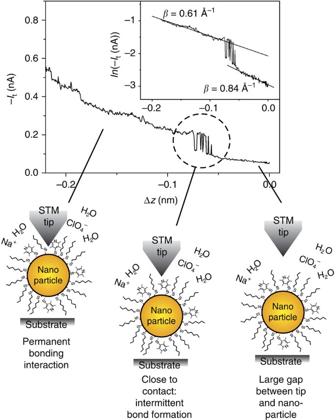Figure 2: Switching behaviour in an electrode/nanoparticle/electrode junction. The STM tip approaching a layer of Au145nanoparticles on Pt(111); switching becomes apparent at Δz∼−0.06 nm. At first, there is no direct chemical interaction between the tip and the particle and the tunnelling current low (right). However, in a small distance range, chemical bonds are formed and immediately disrupted, most likely due to spatial constraints and drift of the STM tip relative to the sample (centre). Finally, the tip/particle distance is small enough that bonding interactions are established permanently; the tunnelling current no longer fluctuates. Inset: The same plot on a semi-logarithmic scale. The slope is (inversely) proportional to the tunnelling barrier, indicating that the latter is lower when the tip is in contact with the particle coating.Itis the tunnelling current; Δzthe distance change applied to the STM tip with respect to the substrate.βis the decay coefficient. Adapted, with permission, from ref.50. (Copyright 2007 American Chemical Society). Figure 2: Switching behaviour in an electrode/nanoparticle/electrode junction. The STM tip approaching a layer of Au 145 nanoparticles on Pt(111); switching becomes apparent at Δ z ∼ −0.06 nm. At first, there is no direct chemical interaction between the tip and the particle and the tunnelling current low (right). However, in a small distance range, chemical bonds are formed and immediately disrupted, most likely due to spatial constraints and drift of the STM tip relative to the sample (centre). Finally, the tip/particle distance is small enough that bonding interactions are established permanently; the tunnelling current no longer fluctuates. Inset: The same plot on a semi-logarithmic scale. The slope is (inversely) proportional to the tunnelling barrier, indicating that the latter is lower when the tip is in contact with the particle coating. I t is the tunnelling current; Δ z the distance change applied to the STM tip with respect to the substrate. β is the decay coefficient. Adapted, with permission, from ref. 50 . (Copyright 2007 American Chemical Society). Full size image While the molecular origin of the above mentioned tunnelling current modulations are fairly well-understood, the origin of other observed switching phenomena is less clear. For example, Tao and coworkers [25] have observed telegraphic switching events—alternating 'high conductance' and 'low conductance' states—in water-filled tunnelling junctions with characteristic lifetimes in the range of micro- to milliseconds. Interestingly, these fluctuations did not show a significant dependence on solution pH, nature or concentration of the electrolyte, or bias voltage; in contrast, they were strongly affected by the gap width. The authors hypothesized that local electronic states in the tunnelling junction potentially stabilized by the local water structure or image charge effects may be responsible for these fluctuations. While it is very difficult to characterize and establish the molecular origin of these states in the tunnelling junction, the findings are reminiscent of the work of Nitzan and coworkers [16] . However, in their calculations, they found the lifetime of these cavities to be much shorter (10 fs) than the current fluctuations observed by Tao and coworkers [25] ( ∼ μs to ms), so further investigation is clearly needed. Interestingly, similar cavities are predicted to exist in ILs [53] . ILs are composed entirely of ions and are thus salts with melting points below 373K. Relative to water, they tend to be rather viscous, suggesting that such cavities may have longer lifetimes, perhaps long enough to be detected directly by tunnelling current modulation. Indeed, relatively large current fluctuations have been observed in an IL-filled single-molecule junction, but were not discussed explicitly [54] . It is interesting to speculate whether such states have a role as intermediates in interfacial charge transfer processes in general or whether they are 'tip-induced' and thus specific to the nanogap configuration. The idea of probing catalytic reactions by tunnelling is in some way a logical progression from earlier work on characterizing interfacial redox processes at the single-molecule level. Such effects were predicted theoretically by Ulstrup, Kuznetsov, Schmickler and others [55] , [56] , and then observed experimentally first by Tao [57] for iron porphyrin and by others [58] , [59] , [60] . Kuznetsov also recognized the discrete, stochastic nature of redox-mediated tunnelling and the relation to fundamental properties of the charge transfer process [61] , [62] , but experimental data are not yet available. Such redox-mediated tunnelling modulations are by no means restricted to small redox molecules, and have also been detected for redox proteins, such as cytochrome c and azurin, and even redox enzymes under catalytic reaction conditions [27] , [63] , [64] , [65] , [66] . Detecting catalytic reactions by tunnelling, say in an (electrochemical) STM setup, has interesting prospects. First, the high spatial resolution of the technique in principle allows probing chemical reactivity at the single-molecule (catalyst and enzyme) level and 'reactivity mapping' across the surface: the stronger the contrast modulation in an STM image, the more active the catalyst. Alternatively, one could probe an individual catalyst molecule or enzyme over time, which is technically possible even at room temperature and in solution [67] . Provided the temporal resolution of the measurement is high enough, individual catalytic turnover events could be detected as modulations (or bursts) in the tunnelling current. Hence, the activity of a single enzyme could be monitored over time to establish whether it undergoes 'sleep and work' cycles, as suggested for some enzymes in solution [68] , or whether all enzymes on the surface are equally active. This is currently unknown and there is probably no technique available at present that could provide this information for non-fluorescent, surface-immobilized species. Catalytically modulated tunnelling may occur when at least two states of the catalyst have sufficiently different tunnelling conductance. An example is the 'open' state of an enzyme E with tunnelling conductance G E (no catalytic substrate molecule S is bound) and bound state ES with conductance G ES , Fig. 3 . We shall assume G ES > G E for the argument's sake here. The scheme below shows a simple Michael–Menten-type enzymatic process, including a fast regeneration step of the catalytic centre. 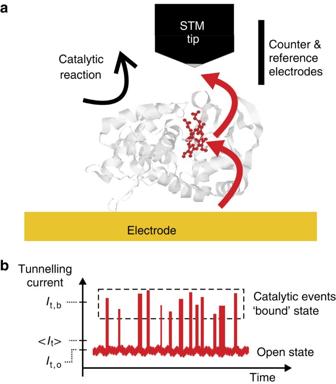Figure 3: 'Catalytic' tunnelling current modulation induced by chemical reactions at the catalytic centre. Cytochromecperoxidase (pdb accession code:2CYP) is taken as an example here, but other 'reactive' molecular bridges would cause the same effect provided different states during the reaction have different tunnelling conductance. Electrons tunnel from the electrode to the STM tip (red arrows), mediated by the catalytic centre (here: heme). Catalytic turnover takes place at the same time (black arrow), which modulates the tunnelling conductance of the enzyme and hence the tunnelling current. The effect is illustrated for a simple two-state system ('open' versus 'bound') in (b), but more complex schemes, where different intermediates have different tunnelling conductance are conceivable. Figure 3: 'Catalytic' tunnelling current modulation induced by chemical reactions at the catalytic centre. Cytochrome c peroxidase (pdb accession code: 2CYP ) is taken as an example here, but other 'reactive' molecular bridges would cause the same effect provided different states during the reaction have different tunnelling conductance. Electrons tunnel from the electrode to the STM tip (red arrows), mediated by the catalytic centre (here: heme). Catalytic turnover takes place at the same time (black arrow), which modulates the tunnelling conductance of the enzyme and hence the tunnelling current. The effect is illustrated for a simple two-state system ('open' versus 'bound') in ( b ), but more complex schemes, where different intermediates have different tunnelling conductance are conceivable. Full size image In the single-molecule regime, probabilities replace the concentrations of reactants in the respective rate equations [69] . The reaction rate is now the probability of turnover from the initial state to product formation with a waiting time distribution f ( t ) that depends on all rate constants and the substrate concentration. For enzymes, the time between individual events is typically on the order of μs to ms, which is slow compared with the rate of tunnelling charge transport. Hence, many electrons are transferred while the catalyst is in a given state, say 'E' or 'ES', with mean lifetimes of τ E and τ ES . STM imaging is, however, relatively slow and measured currents are a 'long time' mean, averaging out any short-term modulations. Ignoring E′ due to the fast back conversion to E, the mean tunnelling current during the catalytic process is then: However, the difference between G ES and G E is unlikely to be drastic, say G ES =1.1· G E , and τ ES =1/10· τ E . The effective, steady-state change in tunnelling conductance due to enzymatic activity is then only ∼ 1%; this is difficult to detect, especially given other sources of interference such as Faradaic processes. On the other hand, if the tunnelling current modulation is measured as a function of time at high resolution, a telegraphic noise pattern is expected to emerge due to switching between E and ES. The effect is roughly one order of magnitude larger ( G ES / G E ) and resolved more easily. Moreover, it is then possible to extract waiting time distributions directly, giving access to kinetic and mass transport parameters at the single-enzyme level, as well as information about the tunnelling process itself (from the amplitude). The effect of the presence of tip on enzyme activity would have to be explored, as well as its influence on the mass transport properties of substrate S towards the catalytic site as well as of the product P away from it [70] . Obviously, the same rationale applies to more complex reaction mechanisms [69] . There are a number of examples where such catalytic effects have been detected in STM imaging, both for small metal complexes and redox enzymes. Hulsken et al . studied monolayers of manganese porphyrin on gold surfaces immersed in n -tetradecane—so in liquid environments but not under 'electrochemical' conditions [26] . In the presence of dioxygen, this metal complex catalyses the conversion of cis -stilbene to cis -stilbeneoxide involving Mn(IV). Interestingly, while in the absence of O 2 , the STM contrast remains somewhat uniform across the monolayer, meaning that all catalyst molecules have more or less the same, relatively low tunnelling conductance. When the concentration of O 2 is increased, however, more and more catalyst molecules 'lighten up' implying that their tunnelling conductance becomes larger. This shows that catalytic activity can not only be detected in this way, but also resolved with molecular resolution. The study of even small enzymes by STM in solution is difficult, as they are already 'large' by tunnelling standards ( ∼ 2–3 nm). On the other hand, solution environments are required, in order to preserve the enzyme's structure and functionality. Tunnelling modulation may therefore be expected to be less prominent than in the Mn porphyrin case above. Ulstrup et al . were the first to demonstrate the effect of enzymatic activity on STM imaging for cytochrome c nitrite reductase ( E. coli ), which is a multi-haem redox enzyme that reduces nitrite to ammonium [28] . Presence and catalytic activity of the enzyme on the electrode surface was confirmed by monolayer voltammetry. Statistical analysis of electrochemical STM imaging data in the absence and presence of catalytic substrate (nitrite) showed that the apparent height of the enzyme decreased in the presence of nitrite. This suggests that the average molecular tunnelling conductance is in fact decreased during the catalytic reaction, that is, the 'bound' state should have a lower tunnelling conductance than the inactive, 'open' state. Some caution needs to be exercised when interpreting the results, however: First, the apparent height of the enzyme is only an indirect measure of the tunnelling conductance. It is determined relative to the surrounding electrode surface. If in the presence of nitrite, Faradaic processes cause a measurable background current, then this reference level may increase and the enzyme appears in effect smaller. Faradaic effects were considered explicitly in similar experiments on glucose oxidase by Stimming et al . [27] Second, as discussed above, the distance dependence of the tunnelling current can be rather complex. Ensuring that the tunnelling current measurement in an STM configuration taking place at the same tunnelling distance in both cases is rather challenging, unless additional structural information is available, for example, from concurrent force measurements [66] . Third and as discussed above, given that the steady-state tunnelling current is weighted mean of the individual tunnelling current modulations, the contrast change during imaging is likely to be smaller than the true difference between the putative conductance states. This is particularly so, when binding events are rare (that is, due to low solution concentrations of the catalytic substrate or hindered mass transport to the catalytic centre) and the lifetime of the 'bound' state is short compared with the open state. In summary, it appears that significant progress has been made towards studying catalytic and enzymatic processes at the nanoscale using tunnelling-based methods. The dynamics of these processes, in terms of temporal fluctuations and 'catalytic noise' in the tunnelling current, have not been addressed to date, but potential applications may arise in small-molecule sensing, for example. The idea of using of STM to sequence DNA emerged soon after the invention of the technique, when sub-molecular resolution images of DNA on various substrates and in various media became available [34] , [35] , [71] . It is essentially based on the characteristics of the tunnelling current discussed above, namely the strong distance dependence and electronic sensitivity of the tunnelling effect. That would in principle enable the technique to differentiate different bases, even when they are located next to each other in a DNA strand. Importantly, 'sequencing-by-tunnelling' would not necessarily require any labelling, which adds significantly to the cost of competing sequencing technologies using fluorescent or radioactive tags. Moreover, it would not be restricted to DNA—once implemented, it could also be applied to other (bio)polymers, such as RNA or peptides/proteins, and even to detect modified bases for epigenetic profiling. The capability to detect and differentiate (all four) DNA bases does not make tunnelling a competitive and commercially viable sequencing technique. Not only has sequencing-by-tunnelling to be feasible, it must also compare favourably with established and 'next-generation', single-DNA sequencing technologies, in terms of error rate, speed and cost [72] . Ideally, such a technique should also be easy-to-use (that is, potentially by a non-expert user) and not require sophisticated laboratory environments. Although this is not the case for DNA sequencing by STM, the latter does establish the foundations of any future tunnelling-based sequencing technique. Recently, these efforts have gained new momentum, especially with the advent of 'personalized genomics' and continued efforts to push the cost of sequencing (a whole genome) to below $1,000 [73] . To this end, one important pre-requisite is to integrate tunnelling-based detection with high-throughput platforms, to optimize sample preparation, handling and, most importantly, speed. Such platforms may be based on solid-state nanopore devices, mechanical break-junctions or nanofluidic structures [74] , [75] , [76] , either on a single device level or (ideally) in a multiplexed format. In contrast to the STM configuration, where the DNA is more or less fixed on the substrate surface and the tunnelling probe (STM tip) is moved over the sample, the tunnelling junction is now fixed and the DNA sample moved across the tunnelling sensor, cf. Fig. 1b . Di Ventra and coworkers [77] , [78] , [79] were the first to investigate theoretically whether the sequencing of single-stranded DNA could be performed by a tunnelling junction aligned with a nanopore, both in a two-electrode and in a four-electrode configuration. The four-electrode configuration was suggested to exert a transversal electric field on the translocating DNA and control the speed and geometric orientation of the strand. They concluded that sequencing should be possible and also investigated the effect of water and other environmental factors including dynamics, as well as tunnelling noise characteristics on the device performance [80] , [81] . Fuentes-Cabrera and coworkers [82] , [83] stressed that in off-resonant tunnelling regime dynamic effects, such as Brownian motion and the exact geometry of the DNA in the junction, may dominate the tunnelling current, rather than base-specific electronic factors. In essence, however, it has become clear that motion of DNA in the tunnelling junction and in particular the DNA/electrode interaction would have to be controlled carefully to make sequencing-by-tunnelling in nanopore configuration a reality. This could be achieved by introducing a second set of transversal electrodes [77] or specific chemical recognition elements or 'chemical adapters' [45] , [47] , [48] , [84] . The key idea of the latter is that when a DNA base enters the tunnelling junction—either as an individual base or in a strand—the chemical adapters bind via hydrogen bond formation, providing a well-defined tunnelling pathway, Fig. 4 . 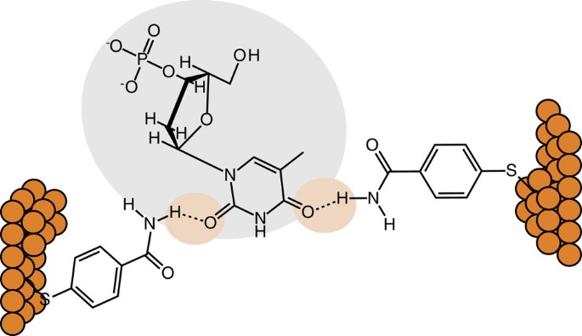Figure 4: Hydrogen bonding can facilitate base recognition. Shown for mercaptobenzamide as recognition element (surface modifier) and thymine monophosphate (grey background). The electrode surface may be rough on the atomic scale, which leads to some variation in surface/molecule electronic coupling—and hence in tunnelling conductance of the bridge. Hydrogen bonding (highlighted in light red) may potentially occur to other parts of the nucleotide, too, for example, the sugar phosphate substituent. Further investigations of the molecular details of this interaction are clearly needed. Figure 4: Hydrogen bonding can facilitate base recognition. Shown for mercaptobenzamide as recognition element (surface modifier) and thymine monophosphate (grey background). The electrode surface may be rough on the atomic scale, which leads to some variation in surface/molecule electronic coupling—and hence in tunnelling conductance of the bridge. Hydrogen bonding (highlighted in light red) may potentially occur to other parts of the nucleotide, too, for example, the sugar phosphate substituent. Further investigations of the molecular details of this interaction are clearly needed. Full size image Interestingly, there is now experimental evidence that all four DNA bases (either as a nucleotide or nucleoside) can be distinguished by tunnelling with good statistical confidence using such an approach [85] . The differences in tunnelling conductance are on the order of several 10 s of pS. This can easily be detected at low speed (small bandwidth of the detection electronics), but may become a significant hurdle for high-speed detection, due to the increasing background electric noise. Again, high-speed detection is an absolute must, if tunnelling-by-sequencing is ever to become a truly competitive sequencing technology. To this end, it seems that the development of customized integrated electronics offers significant potential. For example, Gierhart et al . [33] could resolve low-nA transient nanopore translocation signals in the microsecond range, which indicates that tunnelling-based differentiation of DNA bases may eventually be feasible at kHz rates from an electronics point of view. Tunnelling-based detection is also capable of differentiating methylated from non-methylated cytosine, even in small oligomers [46] , [86] . Methylation patterns in DNA are important for regulating gene expression and provide information about the disease state of a cell (epigenetics) [87] . Unfortunately, these patterns are generally lost during PCR amplification, even though there are some workarounds. In methylation-specific PCR, for example, unmethylated CpG islands are first converted to UpG by bisulphate treatment and then amplified by standard PCR. Hence some information on DNA methylation can be obtained, even though true single-DNA sequencing avoiding PCR altogether would clearly be advantageous. Apart from the detection aspect, however, trying to avoid PCR also poses challenges to sample preparation, especially in a biomedical context where realistic samples usually contain a plethora of different DNA fragments and other biomolecules at comparable concentrations. Amplification provides a means to increase the concentration of the analyte in question, relative to any other 'unwanted' species, and to improve the signal-to-noise ratio. Nanofluidic channels such as solid-state nanopore devices are a very promising route towards implementing a high-throughput tunnelling-based sensing or sequencing platform. With the help of an applied electric field, the nanopore itself forces the DNA (both single- and double-stranded) into a linear configuration, which facilitates tunnelling readout [73] . The read length is potentially much larger than in any other 'third-generation' DNA-sequencing technologies [72] and could potentially exceed several kilobases—if the conformation of such long biopolymers can be controlled. Finally, the operation itself does not require any sophisticated laboratory environments. A solid-state nanopore chip device is about 5 mm by 5 mm in size; sample handling and preparation can be performed in lab-on-a-chip environments; CMOS-based detection electronics could be very small; however, data analysis still requires significant resources. The ultimate speed of such a technology is difficult to assess at this point, because it is not only determined by the actual readout process. Lindsay and coworkers [47] , [48] have estimated the possible read rate to be on the order of 10 bases, based on an estimate of the residence time of the bases in their tunnelling junction, the statistical confidence level required to assign the identity of a base and the translocation force in the nanopore obtained in the previous work by Keyser et al . [88] and van Dorp et al . [89] Note that the force measurements by Keyser et al . [88] were performed on double-stranded λ-DNA, and not single-stranded oligonucleotides used in the Lindsay experiment. This may change the magnitude of the force, but is unlikely to change the qualitative picture. Apart from the readout process itself (and DNA sample preparation and handling), a DNA molecule has to first diffuse towards and enter the nanopore. This is a stochastic process, which depends on the DNA solution concentration and the properties of the nanopore. It also affects the orientation of the DNA strand entering the pore (3′ versus 5′ end). Whereas too low concentrations lead to very small translocation frequencies, too high concentrations result in DNA aggregation and pore clogging. Typical translocation frequencies are on the order of 1–100 Hz. On the other hand, controlling the speed of translocation remains a major challenge [90] , as well as integrating a functional tunnelling junction into the nanopore [75] . Moreover, alignment between the tunnelling-active part and the nanopore is crucial, to avoid DNA by-passing the electrode junction. Designing the chemical adapter is more challenging than in an STM configuration: To bind each DNA base as the strand passes along, the binding kinetics has to be carefully optimized. Strong electric fields inside the nanopore can lead to decomposition of molecular adsorbates and even corrosion of metallic layers on or embedded in the membrane [91] . Finally, careful consideration needs to be applied to the surface chemistry used to bind the adapter to the electrode. Apart from the stability issue, different molecular geometries as well as binding configurations can result in different 'molecular' conductance, depending on the size of the electrode gap. For thiol-based surface modifiers, the differences may be larger than the tunnelling conductance difference between the DNA bases, further complicating data analysis [43] . Other functional groups may be more suitable for this purpose, for example, diazo-based molecules form strong covalent carbon single bonds to gold [92] . Finally, the overall device design needs to be optimized with a view on optimum electric performance, which is, minimizing noise. Integration of the device periphery will help in this respect, but minimizing the effective capacitance of the nanopore chip itself will be equally important. Tunnelling currents have been used in a number of cases for the characterization of interfacial processes in solution and in different contexts. However, a coherent approach to understanding and ultimately exploiting these results is lacking. This is partly rooted in the difficulty of characterizing the tunnelling junction in situ , and partly due to the inherent complexity of such systems. Characteristic tunnelling noise features appear in liquid-filled junctions, which are at least in part due to the local effect of the probe. Existing experimental and theoretical work point towards electronic trap states as a potential origin, but further work is clearly needed to establish the physical basis and structural identity of these states. One could speculate whether such states have a role in interfacial electron transfer processes, particularly in the adiabatic limit when the rate constants are very high and controlled by solvent dynamics rather than electronic coupling. The study of reactive processes in the tunnelling junction, for example catalytically modulated tunnelling, has progressed further in a sense that the molecular event is typically known or can in principle be characterized on a macroscopic level. This is the case in the examples shown above; and catalytic activity has indeed between linked to STM contrast (that is, tunnelling conductance) modulation already. Detection of 'catalytic' tunnelling noise is straightforward from a technical point of view and could also be integrated with STM imaging to provide spatially resolved noise images. Interestingly, such an approach offers unique insight into the reactivity of surface-confined species—such as catalyst or enzymes—at the single-molecule level, even if they are non-fluorescent. The idea of applying tunnelling detection for the analysis of large (bio)polymers, DNA sequencing being a prime example, is very appealing, but also highly challenging. As illustrated in Table 1 and discussed in the previous section, remarkable progress has been made towards fabricating a tunnelling-based sequencing device. Some issues are not easily resolved, but at the same time the potential of high-throughput sequencing-by-tunnelling technology are tremendous. The current state-of-the-art suggests that sequencing of DNA using a tunnelling junction may already be possible, for example in combination with an approach developed by Hagan Bayley and Oxford Nanopore Technologies [93] . In that work, a DNA exonuclease 'upstream' of a molecular recognition element (a cyclodextrin) carefully placed into the opening of a biological pore (alpha-hemolysin). The nuclease cuts an incoming DNA strand into the individual bases, which are then forced down the pore channel by application of an electric field. They then interact with the cyclodextrin and block the pore for characteristic amount of time, allowing read-out of the initial DNA sequence base-by-base ('exonuclease sequencing'). Applied in the present context, the tunnelling detector would have the role of the cyclodextrine, but combined with the sensing ability of the tunnelling current. Such an integrated device has not been implemented to date and hence an estimate of the overall performance is rather difficult. Note that the Oxford team has recently also introduced a new technology that may allow DNA sequencing with an intact DNA strand ('strand sequencing'). Although its performance still has to be fully tested, this could be an important new concept in the sequencing field. Table 1 Developmental stages of a high-throughput DNA sequencing device based on tunnelling detection. Full size table With regards to DNA sequencing, these developments have to be seen against a backdrop of a very competitive DNA sequencing market, which has recently seen the emergence of the first non-optical, massively parallel sequencing device beyond the proof-of-concept stage [94] . Although the base recognition event in the latter technology is at least two orders of magnitude slower than what can be expected from tunnelling-based readout, millions of sensors can be fabricated and operated in parallel. It remains to be seen whether a somewhat more complex tunnelling device can reach similar integration levels. Nevertheless, compositional analysis by tunnelling is not restricted to DNA sequencing alone. Other applications may include the spatially resolved detection of DNA methylation and other epigenetic markers (profiling), the analysis of RNA, peptides or proteins. Although the challenges are tremendous, the opportunities are, too—this promises to be an exciting area of research in the years to come. How to cite this article: Albrecht, T. Electrochemical tunnelling sensors and their potential applications. Nat. Commun. 3:829 doi: 10.1038/ncomms1791 (2012).